A genetic and computational approach to structurally classify neuronal types The importance of cell types in understanding brain function is widely appreciated but only a tiny fraction of neuronal diversity has been catalogued. Here we exploit recent progress in genetic definition of cell types in an objective structural approach to neuronal classification. The approach is based on highly accurate quantification of dendritic arbor position relative to neurites of other cells. We test the method on a population of 363 mouse retinal ganglion cells. For each cell, we determine the spatial distribution of the dendritic arbors, or arbor density, with reference to arbors of an abundant, well-defined interneuronal type. The arbor densities are sorted into a number of clusters that is set by comparison with several molecularly defined cell types. The algorithm reproduces the genetic classes that are pure types, and detects six newly clustered cell types that await genetic definition. Generating a systematic census of neuronal cell types is important in understanding brain function. However, even in the retina, a very well-studied region of the central nervous system, the problem is far from settled. It is widely believed that there exist 20 or more types of retinal ganglion cell (RGC), the sole output neurons of the retina [1] . Responses to visual stimuli indicate that each RGC type transmits the output of a retinal circuit performing a distinct visual function [2] , [3] . Yet, existing catalogues do not agree on the identity or number of RGC types despite intensive attempts. The number of putative types in large-scale studies ranged from 12–22 (refs 4 , 5 , 6 , 7 ). Recent technical advances offer a way towards a solution. Genetic methods have been used to molecularly define some RGC types [8] , [9] , [10] , [11] , [12] . This approach is promising but still incomplete. Serial electron microscopy (EM) has also been used to structurally define cell types [13] . In addition to high spatial precision, EM offers the possibility of completeness, as every neuron in a given volume can be reconstructed. In practice, the approach has been limited so far to relatively small volumes and hence to types of RGCs that are relatively small. Here we show that light microscopy (LM), the oldest technique for structural classification of cell types, can be combined with computational techniques to yield improved spatial precision. Since LM is more easily combined with genetic labelling, and is readily applicable to small and large cells, it is complementary to EM. Our method is based on the spatial relationship of a neuron’s dendrites to arbors of its potential synaptic partners. This contrasts with many traditional approaches to structural classification of neurons, which rely on features that quantify the spatial relations between different features of a single cell [4] , [5] , [6] , [7] . To develop and validate the method, we analyse mouse RGCs. Our method has four components: we use histological and computational methods to reduce the sources of non-biological variability in the samples. We create a global coordinate system, by relating the position of each ganglion cell to the layers defined by the dendrites of a well-defined amacrine cell, the starburst cell. We describe RGC dendrites by a single measure, the arbor density [14] , [15] . We use the arbor density function to perform hierarchical clustering of the cells. These steps alone can not define cell types, because there is no theoretically valid way to know where one should segment the hierarchical tree to define the clusters. We solve this problem by including in our sample several sets of RGCs that were independently defined by molecular genetic means [8] , [9] , [10] , [11] , [12] . For most of these types, the cells share visual response properties as well as molecular attributes. Moreover, their somata form regular mosaics across the retina, a fundamental requirement for a retinal cell type. These sets therefore serve as the gold standard of unequivocally distinct RGC types. The transgenic strains allow setting of the level at which the final clusters of the whole sample population (defined and unknown cells) are assigned; the criterion is to maximize the purity of clusters formed by the defined cells at that level, at which point the clusters indicated for the unknown cells should also be valid. The results strongly suggest that this is the case. We then use the molecularly defined cells as a test bed for comparing our methods with results from using the classical structural metrics. Finally, we devise a method to test the reproducibility of the method, by systematically withdrawing an individual cell from the population, carrying out the clustering without it and then asking the algorithm to assign the withdrawn cell to one of the clusters (as though the withdrawn cell had been newly encountered). The test cells are assigned to the proper clusters with very high accuracy. Interestingly, our imaging, registration and classification methods reveal an unexpected level of precision (that is, submicron) in the laminar organization of RGCs using LM. This precision is so pronounced that the full laminar description is enough to distinguish between many (but not all) cell types in a highly heterogeneous data set. Imaging the tissue without conventional mounting We assembled a data set of 363 mouse RGCs drawn from 10 transgenic lines. Seven of these lines (JAM-B [8] , CB2 (ref. 9 ), W3 (ref. 12 ), BD [12] , W7 (ref. 12 ), Cdh3 (ref. 16 ) and K included one or a few genetically defined cell types (see Methods for details of selection. Only bright W3, On Cdh3 and On K cells were used. We identified a very rare (<2%) type in the BD strain, and named the dominant, On–Off direction selective neurons as BDa, the rare subtype as BDb.). In addition to these relatively homogeneous or ‘defined’ lines, three highly heterogeneous ‘at-large’ lines (GFP-M, YFP-H and YFP-12) were included [17] . Each of these lines includes a broad sample of different RGC types [1] , [6] , and the use of three independent genetic lines further extends their potential sample of cells. Following antibody staining and/or microinjection, individual whole-mounted RGCs were imaged by confocal microscopy. We also imaged starburst amacrine cells in a different colour channel. Starburst dendrites arborize in two thin strata of the inner plexiform layer and are stained by antibodies to choline acetyltransferase [18] . We enhanced the image quality of the stacks by using machine-learning-based algorithms. After enhancement, RGC arbors were skeletonized semiautomatically. The starburst layers were automatically detected in the other channel (Methods and Supplementary Figs 1,2 ). We found that conventional mounting deformed the tissue substantially. We minimized this source of error by placing spacers between the coverslip and the slide. Without the pressure of the coverglass, the tissue assumed a wavy form under the microscope. To compensate for curvature and thickness variations of the inner plexiform layer, we digitally unwarped the tissue. We computed a nonlinear transformation that approximately preserved local angles and global distances, and mapped the starburst sublayers into flat planes at fixed depths in the inner plexiform layer [19] , [20] ( Fig. 1 ). The same transformation was applied to the other colour channel, registering the RGCs to a common coordinate system. Notably, this registration involved the use of dendrites and not somata as fiducial markers. Quantitative slope analysis (Methods and Supplementary Fig. 3 ) shows that arbors of individual RGCs are indeed aligned parallel to the starburst amacrine layers by the method. 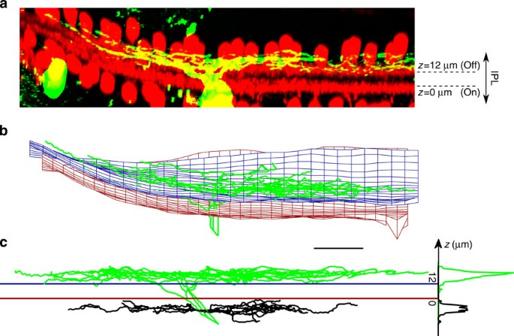Figure 1: Warping neurons using dendritic fiducial markers (a) Side projection of an image stack. Partial RGC (green) and starburst amacrine cell (red) channels merged. (b) The detected dendritic arbor (green) and starburst sublayers (meshes) of the cell in (a). The red (On, bottom) and blue (Off, top) meshes have opaque white faces. Extents of the meshes were chosen slightly differently for visualization. (c) Dendritic arbors (left) and stratification profiles (right) of two RGCs, which were imaged in two different stacks and registered to each other using the On (red) and Off (blue) starburst planes as landmarks. The stratification profile of a cell is its distribution of dendritic length across the depth of the inner plexiform layer. This one-dimensional function is useful in visualizing the cell’s laminar positioning. The green RGC is the result of a nonlinear transformation of the RGC in (a) that flattened the starburst surfaces. The black RGC was obtained by a similar procedure from another image stack. Scale bar, 40 μm. Figure 1: Warping neurons using dendritic fiducial markers ( a ) Side projection of an image stack. Partial RGC (green) and starburst amacrine cell (red) channels merged. ( b ) The detected dendritic arbor (green) and starburst sublayers (meshes) of the cell in ( a ). The red (On, bottom) and blue (Off, top) meshes have opaque white faces. Extents of the meshes were chosen slightly differently for visualization. ( c ) Dendritic arbors (left) and stratification profiles (right) of two RGCs, which were imaged in two different stacks and registered to each other using the On (red) and Off (blue) starburst planes as landmarks. The stratification profile of a cell is its distribution of dendritic length across the depth of the inner plexiform layer. This one-dimensional function is useful in visualizing the cell’s laminar positioning. The green RGC is the result of a nonlinear transformation of the RGC in ( a ) that flattened the starburst surfaces. The black RGC was obtained by a similar procedure from another image stack. Scale bar, 40 μm. Full size image We represented the shapes of RGCs by an arbor density representation [15] , [21] that does not use axial low-pass filtering ( Supplementary Note 1 and Supplementary Fig. 4 ). This three-dimensional (3D) representation was computed by convolving the registered dendritic arbor skeleton with a blurring kernel in the xy directions only, and normalizing (Methods). Crucially, no blurring was applied to the z direction, in order to preserve the laminar structure ( Fig. 2 ). The arbor density implicitly includes many traditional structural features (for example, stratification depth, arbor width and shape), while it discards others (for example, tortuosity and branch angle). 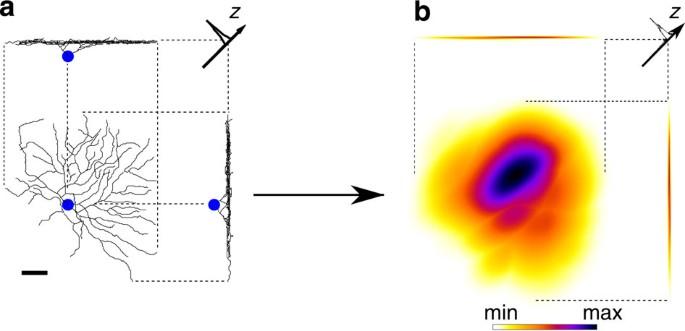Figure 2: Obtaining an arbor density representation for a cell. (a) The lateral and axial projections of a dendritic arbor, along with its stratification profile. Blue dots, approximate locations where arbors attach to cell bodies (not shown). Scale bar, 40 μm. (b) The lateral and axial projections of the arbor density, obtained from the dendritic arbor by anisotropic in-plane blurring. Figure 2: Obtaining an arbor density representation for a cell. ( a ) The lateral and axial projections of a dendritic arbor, along with its stratification profile. Blue dots, approximate locations where arbors attach to cell bodies (not shown). Scale bar, 40 μm. ( b ) The lateral and axial projections of the arbor density, obtained from the dendritic arbor by anisotropic in-plane blurring. Full size image Clusters match with available genetic information The registered arbor density of each cell was represented by a 20 × 20 × 120 ( x × y × z ) image, and read into a 48,000-dimensional vector. The dissimilarities between cells were quantified by the Euclidean distances between their vector representations, and a hierarchical clustering dendrogram was obtained. The amount of in-plane blurring and the cutting level of the dendrogram were chosen so as to minimize the splits and mergers (total confusions—see Methods) of the known genetically defined strains, ignoring their possible subtypes. The data set was divided into 15 clusters ( Fig. 3a and Supplementary Fig. 5 ). Four genetic classes (W3, Cdh3, CB2 and J) were each assigned to single clusters. The algorithm distinguished between W7a, mostly in the middle inner plexiform layer, and W7b, mostly in the outer inner plexiform layer. W7a and W7b correspond roughly to the two subtypes defined previously [12] . The algorithm confirmed the BDb type and assigned those cells and W3 cells to the same cluster. Their stratification profiles are very similar, extending even to the unusually long tail to the right of the peak ( Fig. 4 ). The most likely explanation is that the BDb and W3 appear in two genetically different mouse strains but are indeed the same cell type. Finally, the On cells belonging to the K strain were classified in two different clusters, even though the algorithm had as a criterion minimizing splits of cells from genetically defined lines. 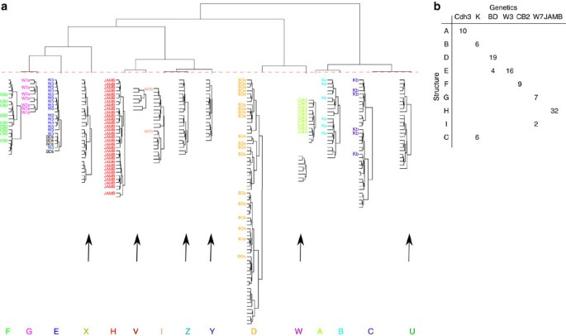Figure 3: Classification using registered arbor densities reveals the matching between genetic and structural cell types. (a) Hierarchical clustering of all the cells in the data set. Individual clusters were rotated for a vertical display and scaled up 7.5 times to reveal the details. Each leaf corresponds to a cell. Cells (leaves) from known genetic strains are labelled while unlabelled leaves correspond to at-large cells. (bottom) Each structural cluster is assigned a capital letter. Arrows indicate putative new cell types. (b) Matrix illustrating the consistent sorting of genetically defined cells into structural clusters. Only nonzero entries are shown. Figure 3: Classification using registered arbor densities reveals the matching between genetic and structural cell types. ( a ) Hierarchical clustering of all the cells in the data set. Individual clusters were rotated for a vertical display and scaled up 7.5 times to reveal the details. Each leaf corresponds to a cell. Cells (leaves) from known genetic strains are labelled while unlabelled leaves correspond to at-large cells. (bottom) Each structural cluster is assigned a capital letter. Arrows indicate putative new cell types. ( b ) Matrix illustrating the consistent sorting of genetically defined cells into structural clusters. Only nonzero entries are shown. 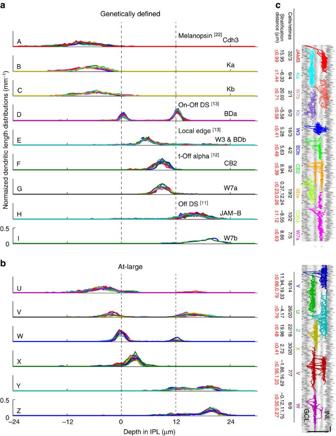Figure 4: Automated clustering of RGCs into 15 types reveals submicron reproducibility of inner plexiform layer depth within each type. Normalized stratification profiles of genetically defined cells sorted by their structural clusters (a) and at-large cells forming new structural clusters (b). Each curve corresponds to a single neuron. The dendritic length of each neuron (area under curve) is normalized to unity. Type E consisted of both W3 (dashed) and BDb cells (solid). Known functional attributes of genetically defined cells are indicated on the corresponding plots. The On and Off starburst planes are located at 0 and 12 μm, respectively. The ganglion cell layer (GCL) is located to the left and the inner nuclear layer (INL) is located to the right. (c) Stratification properties of all 15 types. Stratification distance refers to the distance of peak stratification plane to the ON starburst layer. Images of the cells are not aligned with the profiles—refer to the labels instead. Scale bars, 40 μm. Full size image Figure 4: Automated clustering of RGCs into 15 types reveals submicron reproducibility of inner plexiform layer depth within each type. Normalized stratification profiles of genetically defined cells sorted by their structural clusters ( a ) and at-large cells forming new structural clusters ( b ). Each curve corresponds to a single neuron. The dendritic length of each neuron (area under curve) is normalized to unity. Type E consisted of both W3 (dashed) and BDb cells (solid). Known functional attributes of genetically defined cells are indicated on the corresponding plots. The On and Off starburst planes are located at 0 and 12 μm, respectively. The ganglion cell layer (GCL) is located to the left and the inner nuclear layer (INL) is located to the right. ( c ) Stratification properties of all 15 types. Stratification distance refers to the distance of peak stratification plane to the ON starburst layer. Images of the cells are not aligned with the profiles—refer to the labels instead. Scale bars, 40 μm. Full size image Overall, the defined cells were contained in nine structural clusters labelled by ‘A’ through ‘I’. These clusters display homogeneity and specificity (see below), with little mixing across cells from molecularly defined strains. The matching matrix of Fig. 3b shows only three nonzero off-diagonal elements, indicating that cells of two structural types are rarely assigned to one genetic class, and vice versa . Although the number of clusters and the amount of filtering were optimized, a few off-diagonal elements persisted because of heterogeneity within or overlap between some genetic classes, as explained above. Of the 252 ‘at-large’ cells, 141 were assigned by the clustering algorithm to the same nine structural types as the ‘defined cells.’ The remaining 111 at-large cells were assigned to six structural types that included no genetically defined cells, and were given the provisional names U, V, W, X, Y and Z. These six types represent new cell types that await future molecular definition. Precision in laminar organization Figure 4a and Supplementary Fig. 6 show the stratification profiles of the defined cells, sorted by their structural types, and also by the genetic classes to which they most closely correspond. It should be kept in mind that clustering was performed based on the complete arbor density; stratification profiles are only used as a convenient means of visualizing the results of clustering. Nonetheless, it is notable that for many of the cell types, the s.d. of the stratification peak was ⩽ 1 μm ( Fig. 4c ). As an example, the profiles of the W3 cells were highly stereotyped and the s.d. of the profile peak location was 0.41 μm. Even that striking statistic, however, does not do full justice to the stereotypy, which extends to the entire shape of the profile, including the long tail to the right of the peak. Some types in Fig. 4a have very similar normalized stratification profiles. They are clustered separately, however, because the algorithm makes full use of the registered arbor density. Thus, although stratification level is a prime determinant of cell type in our scheme, it is not the only determinant. For example, a clean separation between W7a and CB2 is visualized by projecting their 48,000-dimensional arbor density vectors onto the subspace defined by two principal components of the data ( Supplementary Fig. 7a ). This difference is intriguing, as ongoing efforts show that these two types share several physiological and molecular properties. Similarly, Cdh3, Ka and Kb have similar stratification profiles, but look well separated when their arbor densities are projected onto two principal components ( Supplementary Fig. 6 , Supplementary Fig. 7b ). Figure 4b shows the normalized stratification profiles of the cells in the six structural types comprising only at-large cells (U, V, W, X, Y and Z). Again, the profiles are very similar within each type and this is also reflected in the s.d. values of the stratification peak ( Fig. 4c ). We reiterate that cells were registered in depth using an external landmark, the planes of starburst dendrites; they were not registered to each other. Therefore, the cells have more than similarly shaped profiles; their positions relative to the rest of the neurons are highly precise. Previous morphological classification literature is likely to have come across cells of these types. However, a direct comparison is hampered by either the high variability in stratification or incomplete arbor characterizations in those publications ( Supplementary Figs 8 , 9 and Supplementary Note 1 ). One test of the classification scheme was provided by examination of the at-large cells assigned to clusters that include genetically marked types. For example, the two at-large cells assigned to the JAM-B cluster displayed the asymmetric dendrites that were typical of the genetically defined JAM-B cells [8] , even though asymmetry was not an explicit criterion for classification ( Supplementary Figs 10–26 ). Indeed the at-large cells clustered with each of the nine genetic types are similar to their genetically defined counterparts. Supplementary Fig. 7 shows that the statistical properties of each type change little when the at-large cells are added to the defined cells. Note that this did not have to be the case. As an example, the CB2 and W3 cells are laminar ‘neighbours’ in our data set. Their stratification peak s.d. values are 0.39 and 0.41 μm, respectively. Yet, a cluster made up of their merging would have a s.d. value of 1.84 μm. As a further demonstration, we added axial noise only to the at-large cells, and found out that this can destabilize the clusters, result in splits of genetically defined subpopulations and increase the s.d. values (Methods and Supplementary Fig. 27 ). Our observed reproducibility of stratification depth exceeds that of previous attempts, in some cases by an order of magnitude of 4–7 ( Supplementary Fig. 8a ). In relative terms, a s.d. of 0.5 μm corresponds to ~1% of the inner plexiform layer depth. For a comparison with cells’ depth spans within the inner plexiform layer, we measured the minimal depth span that contains 95% of an RGC’s dendritic length. A s.d. of 0.5 μm corresponds to 2–3% of this effective depth span ( Supplementary Fig. 8b ). Finally, the observed laminar precision tended to decrease with increasing distance from starburst layers ( Supplementary Fig. 28 ). Variability in lateral dendritic pattern The sensitivity and specificity in laminar organization contrasts with the variability in lateral morphology (that is, in the cells’ morphologies as seen in the usual whole-mount view). 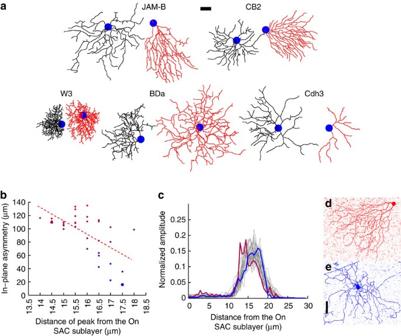Figure 5: Strongly defined genetic types can nonetheless display high variability in their tangential profiles. (a) Projections of selected JAM-B, CB2, W3, BDa and Cdh3 cells onto thexyplane. For a complete view of every cell of each type, seeSupplementary Figs 11–26. (b) Asymmetry versus position of peak stratification shows a negative correlation for JAM-B cells. Asymmetry was quantified by the distance between the centre of mass of a skeleton and the node representing the soma. The most asymmetric cell is represented by pure red and the most symmetric cell is represented by pure blue. The remaining cells are coloured according to their asymmetry values, by a linear combination of red/blue (relative asymmetry/symmetry). (c) Red and blue stratification profiles correspond to large red and blue circles in (b) and asymmetric and symmetric cells in (d,e) (these differences are known to reflect different physiologies—see text). Scale bars, 40 μm. Figure 5a displays whole-mount views of selected cell pairs from the strongly defined types; JAM-B, CB2, W3, BDa, Cdh3 ( Supplementary Fig. 10 shows the corresponding raw fluorescence images). These classes represent homogeneous cell types because they share basic structural, molecular and, in most cases, physiological properties. Yet, their xy views appear quite variable. Supplementary Figs 11–26 display the whole-mount views of all the cells in the data set sorted by their clusters, and demonstrate the full range of shape variation, despite the great stereotypy shown in Fig. 3 . Figure 5: Strongly defined genetic types can nonetheless display high variability in their tangential profiles. ( a ) Projections of selected JAM-B, CB2, W3, BDa and Cdh3 cells onto the xy plane. For a complete view of every cell of each type, see Supplementary Figs 11–26 . ( b ) Asymmetry versus position of peak stratification shows a negative correlation for JAM-B cells. Asymmetry was quantified by the distance between the centre of mass of a skeleton and the node representing the soma. The most asymmetric cell is represented by pure red and the most symmetric cell is represented by pure blue. The remaining cells are coloured according to their asymmetry values, by a linear combination of red/blue (relative asymmetry/symmetry). ( c ) Red and blue stratification profiles correspond to large red and blue circles in ( b ) and asymmetric and symmetric cells in ( d , e ) (these differences are known to reflect different physiologies—see text). Scale bars, 40 μm. Full size image In the case of JAM-B cells, we were able to relate one aspect of this variability to the small laminar ‘jitter’. As it turns out, a subpopulation of JAM-B cells at the dorsal and ventral margins of the retina is known to have relatively symmetric dendrites, in comparison to the majority, which have a wedge-shaped dendritic field [8] . The symmetric JAM-B cells are functionally different from the asymmetric ones, as they exhibit less direction selectivity [8] . We found that symmetric cells tend to stratify closer to the inner nuclear layer ( r =−0.62, P =2 × 10 −4 , n =32, t -test; Fig. 5 ) than do asymmetric cells. Even though it is subtle, this slight variation in JAM-B stratification profiles is correlated with a functional property, direction selectivity. Thus laminar variation does not seem to be simply due to measurement noise. It could possibly be developmental variation, or instead a meaningful central-to-peripheral difference in design. In any case, it is a striking example where the cells’ lamination is a more robust feature than the details of their lateral morphology. Traditional structural features are weak classifiers We compared our method to some of the traditional measures that have been used to categorize RGCs morphologically. ( Fig. 6 , Tables 1 and 2 ). Table 1 tabulates the statistics for the strongly defined types in the data set (JAM-B, CB2, W3, BDa and Cdh3). It is immediately apparent that the traditional parameters used are much worse at identifying the known cell types than our algorithm (many other such parameters were devised in previous literature, but they were shown to be heavily correlated with each other, and a few well-chosen parameters captured most of the variation [5] ). 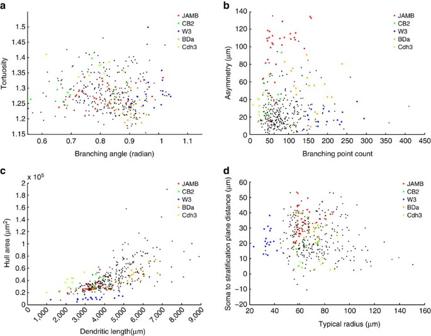Figure 6: Classical features are weak classifiers of cell types. (a–d) 2d plots of various classical features for the five strongly defined types and the rest of the data set (smaller, black dots). Figure 6: Classical features are weak classifiers of cell types. ( a – d ) 2d plots of various classical features for the five strongly defined types and the rest of the data set (smaller, black dots). Full size image Table 1 Means and s.d. values of various classical features for the strongly defined types. Full size table Table 2 Clustering performance of various features due only to the strongly defined types after digital flattening. Full size table To further quantify the lack of sensitivity and specificity of classical morphological features in clustering RGC types, we clustered the whole data set with these alone. Table 2 shows that clusters produced by such features resulted in many misclassifications even in the strongly defined subset. This subset serves as a test bed, where a viable scheme is expected to achieve perfect classification, considering the wealth of full RGC diversity. We also computed the classification performance due to the median z -position, after our registration method was applied. This registered depth metric resulted in a remarkable increase in accuracy when compared with the performance of the soma-to-stratification distance, which is another measure of lamination depth. Note that our imaging and processing methods were instrumental in revealing this increased accuracy compared with previous literature ( Supplementary Fig. 8 ). This result indicates, in line with expectations, that stratification position has an overpowering role in determining RGC identities while it is not enough to explain the full diversity by itself. We sought to combine the median z -position with the dendritic length (a feature of arbor complexity) and typical radius (a feature of lateral extent) parameters by choosing optimal weights. While the result improved, it still produced misclassifications even in this relatively simple task of correctly clustering only the five strongly defined types. Moreover, this classifier discovered only nine clusters over the whole data set and did not perform well in a test of robustness. Prospective testing of the reliability of clustering If the clusters (cell types) are reliable, a newly encountered cell should reliably be assigned to the correct cluster—that is, to the cluster made up of cells of the same type as the new one. We verified this prediction by a ‘thought experiment’ in which the algorithm was confronted by a new cell, but one whose identity we knew. This was done by a leave-one-out analysis ( Fig. 7a ). Each neuron was excluded from the data set in turn. The remaining 362 cells were clustered again, with the cutting level chosen—independent of the original analysis—by the algorithm. The clustering scheme was then confronted with the left-out cell, which was assigned to that cluster whose arbor density mean was closest in terms of Euclidean distance. In other words, the left-out cell was approached as though it were a completely foreign cell (even though we knew from the original clustering which cluster it should belong to). This protocol was repeated for each of the 363 cells. Note that the number of clusters was not restricted. 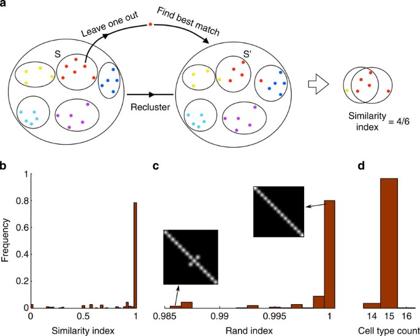Figure 7: Leave-one-out cross-validation suggests that the individual cluster assignments are robust and specific. (a) Schematic of the leave-one-out study. The best match cluster is the newly formed cluster whose cells are structurally most similar to the deleted cell. (b) Distribution of the similarity index over the whole data set. The similarity index is a measure of prospective cell type assignment capability; 0 denoting the worst score and 1 denoting the perfect score (see text). (c) Distribution of the Rand index over the whole data set, showing that reassignment of cell types rarely change after a cell is deleted. Insets: binarized matching matrices generating the lowest and the highest Rand indices, where each row (column) corresponds to a cluster of the original (one-left-out) clustering. A white pixel indicates a nonzero intersection and a black pixel indicates a disjoint cluster pair. (d) Distribution of the discovered number of clusters over the whole data set, demonstrating the effect of taking one cell out on the resulting number of clusters. Reclustering the data set without the left-out cell virtually always resulted in 15 clusters. Theyaxis is common to (b–d). Figure 7: Leave-one-out cross-validation suggests that the individual cluster assignments are robust and specific. ( a ) Schematic of the leave-one-out study. The best match cluster is the newly formed cluster whose cells are structurally most similar to the deleted cell. ( b ) Distribution of the similarity index over the whole data set. The similarity index is a measure of prospective cell type assignment capability; 0 denoting the worst score and 1 denoting the perfect score (see text). ( c ) Distribution of the Rand index over the whole data set, showing that reassignment of cell types rarely change after a cell is deleted. Insets: binarized matching matrices generating the lowest and the highest Rand indices, where each row (column) corresponds to a cluster of the original (one-left-out) clustering. A white pixel indicates a nonzero intersection and a black pixel indicates a disjoint cluster pair. ( d ) Distribution of the discovered number of clusters over the whole data set, demonstrating the effect of taking one cell out on the resulting number of clusters. Reclustering the data set without the left-out cell virtually always resulted in 15 clusters. The y axis is common to ( b – d ). Full size image We measured the clustering accuracy of the left-out cell by comparing the intersection and the union of the two clusters the cell was assigned to (that is, the original cluster and the new cluster formed by the leave-one-out study). We defined the similarity index as the ratio of the intersection set’s cell count and the union set’s cell count, excluding the left-out cell from both sets (Jaccard index of the differences of the two sets from the left-out cell). This index produces a maximum score of 1 when the two clusters are identical, and a minimum score of 0 when the two clusters are disjoint ( Fig. 7b and Supplementary Fig. 29 ). In most cases, the left-out cell was assigned to the identical or a very similar cluster. We also measured the overall similarity by calculating the Rand index [22] between the two different clusterings, once for each instance of the leave-one-out study. The Rand index produces a maximum score of 1 when the two clusterings are identical, and a minimum score of 0 when no cell pair is classified consistently between the two clusterings ( Fig. 7c ). The insets of Fig. 7c display binarized matching matrices corresponding to the instances generating the lowest (0.986) and highest (1, perfect matching) RI values. Finally, since the number of clusters were independently chosen in each instance of the leave-one-out study, we counted the number of clusters ( Fig. 7d ). The count varied between 14 and 16, and it was equal to 15 with >96% frequency (349/363). Thus the number of cell types in the data set and the assignment of individual cells to those types appear to be determined robustly. Supplementary Fig. 30 demonstrates the dynamic range of the reported numbers, the tightness of clusters through a randomization study and the performances of the Σ classifier in Table 2 and a classifier based only on the depth profiles. We describe here an objective method for structural classification of cell types, which tunes itself using both structural and molecular information. Subsequently, new cells can be classified based purely on structural criteria. The sorting into cell types was remarkably precise—as verified by the clean clusters into which molecularly defined cells were sorted—and is reproducible. The observed precision suggests that the conventional division of the inner plexiform layer into only a few sublayers should be refined. In absolute terms, the variability is even smaller than observed in axonal arbors of the fly olfactory system [21] , and much smaller than in the hunchback expression pattern of the fly early embryo [23] . The method depends only on the distribution of the cells' dendritic arbors in space, and it is notable that the simple arbor density representation combined with a spatial system of registration seems to capture much of the relevant structural information in RGCs. As for any classification system, new types obtained in this way will need independent verification. Physiological testing will be important ( Supplementary Note 1 ), and genetic markers should be eventually found for them as well. The decrease in observed laminar precision with increasing distance from starburst layers ( Supplementary Fig. 28 ) can be explained, at least in part, by the use of two fiducial layers as markers. Availability of more neurite-based landmarks outside of the starburst layers may further improve the observed reproducibility. A single stratification value—which can be approximated from flatter parts of a cells’ dendritic arbors—was inadequate to account for the full diversity of RGCs. Combinations of a few explicit features were not sufficient either, and the full arbor density was needed to prevent misclassifications. The low-detail representation of the lateral arbor density was a reflection of the variability in the lateral structures of the dendritic arbors. While this variability may have functional significance, it seems more likely that the lateral spread of the RGC dendrites is under less biological pressure for accuracy than the depth of stratification, which has an overpowering role on the possible connectivity of the cells. Our clustering identifies 15 RGC types. How many more might exist? It has generally been thought that the genetically driven markers in the ‘at-large’ strains are randomly expressed in ganglion cells, though this is far from certain. In attempting a broad survey we collected the at-large cells from three different mouse strains, which express different marker proteins and show different numbers of labelled cells. However, the sample is unlikely to be complete. Although some genetically identified cells may be among our unidentified ‘at-large’ cells (that is, provisional types U, V, W, X, Y and Z), a few known cell types are still missing from our data set. At the least, it is unlikely that our sample includes all types of the sparse melanopsin-expressing cells [24] , [25] . As a purely semantic matter, we are of course unable to identify the four directionally tuned subtypes of On–Off direction selective cells (the BDa cells) and if they are counted as distinct ‘types’ the number would be increased. A complete categorization does seem attainable however with a larger and more systematic sampling of RGCs ( Supplementary Note 1 ). EM complements LM with its superior resolution and promise of solving the sampling problem through reconstructing every neuron in a given volume [13] . These two techniques may integrate further to study cell type-related problems in the retina. Our methods offer a precise way of comparison across different studies ( Supplementary Note 1 ). We also speculate that some of our methods may be applicable to other laminar structures, such as the cortex, while a more direct extension could be to study costratification of (and to classify) neuron classes whose arbors occupy the inner plexiform layer (that is, bipolar, amacrine and ganglion cells). Anaesthesia and retinal extraction All animal procedures were approved by the Research Animal Care Committee of the Massachusetts Eye and Ear Infirmary. Thy1-GFP-M, Thy1-YFP-H, Thy1-YFP-12, K, JAM-B-CreER, BD, W3-YFP, W7-YFP and Thy1-STOP-YFP lines were generated in the laboratory of J.R.S. [8] , [12] , [17] , [26] . Cdh3-GFP and CB2-GFP lines were generated by GENSAT [9] , [16] , [27] ; CB2-GFP retinas were generously provided by Dr A. Huberman (UC San Diego). Animals were 1–6 months old and of both sexes. All animals were anaesthetized with ketamine (30 mg per kg) and xylazine (3–6 mg per kg) and killed by overdose of the same agents and cervical dislocation. Tissue preparation and imaging Retinas were blocked in 5% Normal Donkey Serum with 1% triton in PBS anywhere between 2 hours to overnight prior to antibody incubations. In GFP-M, BD, W7, Cdh3, K, JAM-B and CB2 retinas, the GFP signal was amplified by antibody staining (anti-GFP, Millipore, AB3080P). This step was done for YFP-12 retinas without a permeabilization agent, to reduce the density of labelling. Since CB2, W3, some W7 and some K retinas were densely labelled, individual live cells were microinjected with 0.5% Lucifer Yellow (Invitrogen, L453) and 4% Neurobiotin (Vector Laboratories, SP-1120), followed by streptavidin labelling (1:200 Rhodamine-Streptavidin (TRITC) conjugate, Jackson Immunolabs, 016-020-081). Fixed YFP-12 cells were injected with 1% DiI (Invitrogen, D282) in 100% ethanol, using electrodes backfilled with 100% ethanol. To avoid fixation artifacts, the retina was first removed from the eye to speed up penetration of fixative. In all retinas, starburst amacrine cells were labelled by antibody staining of ChAT (1:1,000 Chat anti-goat followed by 1:500 CY-5 anti-goat, Millipore, AB144). When retinas were mounted for imaging, coverglass fragments were used as spacers between the coverslip and the slide to allow the retina to curve naturally. Images were acquired on an Olympus FV-1000 or a Leica SP5 confocal microscope using a × 40 oil immersion lens, at 12 or 16 bits per voxel, and at a voxel size of 0.4 × 0.4 × 0.5 μm 3 . Image enhancement by convolutional networks Convolutional networks (CNs) were trained to enhance the anti-GFP and anti-ChAT images using the CNPKG software ( http://github.com/srinituraga/cnpkg/ ). The anti-GFP CN was trained to transform noisy greyscale images of neurons into cleaner binary images. Training stacks for backpropagation learning in CNs [28] were obtained by manually skeletonizing the arbors of 21 neurons using KNOSSOS [29] , and expanding the skeletons to match dendrite widths in the original image in a manner that preserved topology [30] . The anti-ChAT CN was similarly trained to enhance noisy images of starburst amacrine dendrite sublayers. CNs had eight feature maps in each hidden layer, with all-to-all connections between successive layers. The anti-GFP CN used six layers of filters with sizes 5 × 5 × 1, 5 × 5 × 1, 3 × 3 × 3, 5 × 5 × 1, 3 × 3 × 3 and 1 × 1 × 1, so that each output voxel was influenced by a 17 × 17 × 5 field of view in the input. The anti-ChAT CN used three layers of filters with sizes 25 × 25 × 3, 25 × 25 × 3 and 1 × 1 × 3, so that each output voxel received input from a 49 × 49 × 7 input field of view. The 25 × 25 × 3 filters were composed of 5 × 5 × 1 patches, each of which was constrained to be uniform. Arbor skeletonization and detection of starburst sublayers Enhanced anti-GFP images of neurons were semiautomatically skeletonized using Simple Neurite Tracer [31] , with an average tracing time of 40 min per cell. Since skeletonization was often challenging due to dense labelling and/or poor image quality, each stack was skeletonized by at least two trained image analysts. The skeletons for each neuron were inspected by one of the authors, and one was chosen for inclusion in the data set. Usually the skeleton with the greatest total dendritic length was chosen, since other skeletons showed evidence of missing branches. However, a shorter skeleton was selected in some cases, as other skeletons contained extraneous branches. Some neurons were excluded altogether, as extensive overlap with other neurons made them impossible to skeletonize accurately. The starburst sublayers were automatically located in enhanced anti-ChAT images by maximum detection. For stacks with poor image quality, starburst sublayers were manually annotated by marking 200–500 irregularly spaced points per sublayer, which took roughly 10 min per stack. Then, two smoothness-regularized least-squares surfaces were independently fit to the corresponding data points as approximations of the two starburst sublayers. Definitions of dendritic arbor features Hull area is the area of the tightest convex hull containing the z -projection of the dendritic arbor (in μm 2 ). Branch point count is the number of branch points within the dendritic arbor. Dendritic length is the total length of the dendritic arbor (in μm). Median branch length is the median dendritic segment length of all the segments starting and ending at irreducible nodes (in μm). Irreducible nodes are the points of the dendritic arbor corresponding to soma, branching points or terminal points. Average angle is the mean of the positive angle between (parent node, node) and (node, child node) vectors, where node, parent node and child node are irreducible nodes (in radians). Average tortuosity is the average value of the ratio of the actual dendritic length to the Euclidean distance between irreducible nodes. Asymmetry is the in-plane ( xy ) distance of the soma node to the dendritic arbor (skeleton) centre of mass (in μm). Soma-to-stratification depth distance is the z -distance of the soma node to the dendritic arbor (skeleton) centre of mass (in μm). Typical radius ( λ ) is the root-mean-square in-plane ( xy ) distance of dendritic arbor points to the centre of mass (in μm). Median z -position is the median z -position of the registered dendritic arbor (in μm). Clustering metrics The number of structural splits is calculated as (the number of structural clusters containing at least one cell from a given genetic cluster)−1. The number of genetic splits is calculated as (the number of genetic clusters containing at least one cell from a given structural cluster)−1. The number of structural confusions is the sum of structural splits over all genetic clusters. The number of genetic confusions is the sum of genetic splits over all structural clusters. The number of total confusions is the sum of structural confusions and genetic confusions. Identical clusterings of a data set achieve 0 total confusions. Silhouette denotes the average silhouette value [32] of a clustering. The silhouette value of a cell is a number between −1 and 1, achieving the maximum value of 1 in the case of a perfectly clustered cell. The reported averages in Table 2 are calculated from only the five strongly defined types, within the data set. We produced different hierarchical classifications of the data set using various traditional features and the e-linkage algorithm [33] . We picked the dendrogram cutting levels to assign cluster memberships such that the total confusions of only the JAM-B, CB2, W3, BDa and Cdh3 cells were minimized within the data set. We repeated the same study using the registered median z -position, to see the effect of registration by comparing results for soma-to-stratification depth distance and median z -position. Finally, it was repeated for an additive combination of dendritic length, typical radius and median z -position features by first normalizing the individual features to have zero-mean and unit norm, and then searching for relative weights for typical radius and median z -position features within the [0.2,10] range with 0.2 steps, to minimize the total confusions. Quasi-conformal warping and registration Each starburst sublayer was quasi-conformally mapped [34] to a plane located at its median inner plexiform layer depth. Direct path distances on the diagonals of each surface were calculated to provide the fixed points of the algorithm. Dijkstra’s algorithm [35] provides the exact minimal path distance. We estimated this number by traversing the 3D surface on the diagonal for computational efficiency since retinal tissue is a smooth structure. In each image stack, the quasi-conformal mappings were constrained to hold constant the xy coordinates of the patch in which both starburst sublayers were the flattest. The mappings were extended from the starburst sublayers to points on the skeletonized arbor by using local polynomial approximations (quadratic in tangential coordinates, linear in the axial coordinate). The transformed skeleton was scaled and shifted in z so as to place the On starburst sublayer at z =0 and the Off starburst sublayer at z =12 μm. Then a rigid body transformation in the xy plane aligned the centroid at the origin and oriented the principal axis (the axis of the skeleton with the smallest moment of inertia) along the (1, 1) direction. Model selection and automated clustering Each registered skeleton was gridded, low-pass-filtered and downsampled in the xy plane to yield a 20 × 20 × 120 voxel arbor density representation with a voxel size of 21 × 21 × 0.5 μm (physical representation size: 420 × 420 × 60 μm). Since cells were oriented along the main diagonal, RGCs whose in-plane extent is as large as ~590 μm could fit in the gridding canvas. Traces were registered in depth ( z ) using a Kaiser–Bessel kernel [36] , and in-plane using nearest neighbour interpolation. The initial 720 × 720 xy grid was decimated and low-pass-filtered by retaining the central 20 × 20 low-frequency components in the Fourier space. Further anisotropic xy filtering was applied by using two Kaiser–Bessel kernels with different parameters along the two diagonals, to utilize the (1, 1) orientation of the cells. The full-width-at-half-maximum values of these 20-tap filters were ~2.7 (skew diagonal) and ~4.3 (main diagonal) for the results reported in this paper. Finally, the 20 × 20 × 120 arbor densities were scaled to have Euclidean norms equal to the total dendritic lengths of each trace. The arbor densities were hierarchically clustered using the e-linkage algorithm based on Euclidean distance [33] . A grid search minimizing the total confusions between structural clusters and genetic lines was used to choose the low-pass filter parameters in the (1, 1) and (−1, 1) directions, and the cutting level (threshold) of the dendrogram. Among solutions with the same number of total confusions, a set maximizing the robustness of the clustering, as quantified by the ratio of the dendrogram heights flanking the threshold value, was used. The dendrogram was cut at a height of 0.034, where the maximum dendrogram height was 1. The same clusters are obtained in the range [0.0335, 0.0381]. Stratification peak detection For cell types where the statistics of a single z -profile peak position is reported (that is, monostratified), the peak position of each cell was simply obtained as the depth value at which the profile achieves its maximum value. For cell types where the statistics of two z -profile peak positions are reported (that is, bistratified), one of the peak positions was obtained in the same way. The second peak position was obtained as the depth value at least 6 μm away (half the distance between starburst layers) from the first peak position, at which the remaining profile achieves its maximum value. Data set curation Our primary goal was to sample the cells present in the various lines as broadly as possible. Because of the variability of gene expression that exists in these transgenic lines, no attempt at a uniformly random sample was made, nor was it possible to include minor (faint and/or rare) types that are sometimes present in the transgenic strains. When possible, we deliberately sought multiple examples of rare types. Cells were excluded for poor labelling, excessive dendritic overlap with other cells, poor recovery of the starburst strata or incomplete imaging. Any subtype with less than two representatives was removed from the data set. The K line labels Off type cells as well, but only the On cells were included. Only the On cells in the Cdh3 line were included as we imaged only two On–Off Cdh3 cells and one of them had damaged starburst sublayers. Only the bright cells in the W3 line were included as it was hard to image the dim cells reliably. As mentioned in the text, we found a cell in the BD line that differed from the predominant type [12] . We called this cell BDb, and searched for other atypical cells of this sort, eventually finding four, which resembled each other. In the BD strain, this type of GFP-expressing cell was very rare (<2%). Simulation of axial noise We shifted only the arbors of at-large cells up or down by the imaging step of 0.5 μm with equal probabilities. Therefore, the expected shift of cluster means is 0. Note that it can put an additional distance of 1 μm between some cells of a given type while bringing some cells of different types closer by an additional 1 μm. After noise was added, the clustering procedure was followed as before, trying to minimize the total confusions due to the genetically defined strains. We ran this experiment 100 times, independently. A relevant cluster for a genetically defined cell type is the cluster that contains the highest number of cells of that type. We monitored the number of defined cells in the corresponding relevant clusters for JAM-B, CB2, W3, BDa and Cdh3 cells. JAM-B, CB2 and W3 cells remained in their corresponding clusters in all runs, while BDa and Cdh3 cells were split into multiple clusters ( Supplementary Fig. 27 ). Slope analysis and the accompanying binomial test To test the hypothesis that flattening the starburst amacrine surfaces flattens the RGC stratifications, we quantified the maximum best-fit-line slopes of RGC stratifications projected onto longitudinal planes. For each cell, the part of the dendritic arbor that is at most 4 s.d.s away in z from the cluster mean was retained. This part was projected to the xz plane to obtain a planar set of points. A least-squares line was fit to this set, weighted by the dendritic length they carry. The dendritic arbor was rotated around the z axis by 3° degree steps, and the procedure was repeated for each rotation. The maximum value of the fitted line slopes was recorded for each cell. For bistratified cells, only one stratification was analysed. ( Supplementary Fig. 3a ). For many cells, this value was close to zero and it was <0.02 for almost all cells except for some JAM-B cells ( Supplementary Fig. 3b,d ), showing that mapping the starburst amacrine surfaces onto planar layers indeed maps the RGC stratifications onto planar laminae, to a first degree of approximation. JAM-B cells being an exception is intriguing since this population is known to be direction-selective. We performed a binomial test: a binary variable denoted whether the maximum slope of a cell is >0.02 or not (1 if larger, 0 else). An event probability P was calculated over the whole data set by counting the number of cells with larger slopes and dividing that count by the number of cells in the data set. For each cell type, the number of cells with larger slopes denoted the observed number of successful outcomes ( s ) and the total number of cells in that cluster denoted the total number of outcomes ( n ). The probability p of observing at least s successful outcomes in n total outcomes was calculated according to the binomial distribution ( Supplementary Fig. 3c ): Randomization studies To demonstrate the dynamic range of the Rand index in our study, we picked an integer n uniformly at random from the set {12,13, … ,18} and assigned random cluster identities from a total of n clusters, at each instance of the leave-one-out study. We repeated this study 100 times. Supplementary Fig. 30a displays the distribution of the mean Rand indices from each run that had an upper bound of ~0.86. Clustering algorithms divide any data set into clusters whether tight (‘real’) clusters exist or not. To demonstrate tightness of the discovered clusters, we created a data set of 363 48,000-dimensional vectors, where each element was picked uniformly at random, and repeated the leave-one-out study for this data set, where the dendrogram was cut to produce 15 clusters at each instance. The average similarity index dropped below 0.1 ( Supplementary Fig. 30b ). We repeated the same protocol for a uniformly random data set of 363 five-dimensional vectors. Many cluster similarity indices were <0.5, even in this very-low-dimensional case. Release of software and data Arbor traces and code used in this paper are included as Supplementary Datas 1–13 . The code is also available online at http://github.com/uygarsumbul/rgc . How to cite this article: Sümbül, U. et al . A genetic and computational approach to structurally classify neuronal types. Nat. Commun. 5:3512 doi: 10.1038/ncomms4512 (2014).